Direct and selective hydrogenolysis of arenols and aryl methyl ethers For valorization of biomass, the conversion of lignin to deoxygenated bulk aromatic compounds is an emerging subject of interest. Because aromatic rings are susceptible to metal-catalysed hydrogenation, the selective hydrogenolysis of carbon–oxygen bonds still remains a great challenge. Herein we report direct and selective hydrogenolysis of sp 2 C–OH bonds in substituted phenols and naphthols catalysed by hydroxycyclopentadienyl iridium complexes. The corresponding arenes were obtained in up to 99% yields, indicating the possible production of arenes from lignin-derived bio-oils. Furthermore, the same catalysts were applied to the unprecedented selective hydrogenolysis of the sp 3 C–O bonds in aryl methyl ethers. Thus, the hydrodeoxygenation of vanillylacetone, a lignin model compound, afforded alkylbenzenes as the major products via triple deoxygenation. For more than half a century, the chemical industry has mostly depended on petroleum as chemical feedstock. Because oil is hydrocarbon with a low oxidation state, various selective oxidation processes have been developed for its conversion to value-added chemicals, such as monomers, solvents and intermediates for bulk and fine chemicals [1] . However, oil is a non-renewable resource, and therefore, emerging attention has been focused on the utilization of biomass as a renewable substitute in the last few decades. Unlike petroleum, plant dry matter is mostly composed of highly oxidized carbon compounds such as cellulose and lignin, which are not very amenable for deoxygenation and subsequent processing into chemical compounds on the market. Thus, the development of an efficient technology involving the chemical reduction of biomass has become a great challenge to attain maximum valorization of biomass [2] , [3] . For the reduction of lignin, a major polymeric component of biomass comprising arenols, alcohols and their ethers, intensive studies have been devoted for the development of efficient catalysts aimed at the upgrading of bio-oils, that is, to break them into a mixture of shorter-fragment liquefied fuels [4] , [5] , [6] . Among the various chemical reduction processes, the use of molecular dihydrogen is the most desirable method because it can be the least expensive and the most atom-economical pathway. However, more attention should be concurrently paid to the conversion of lignin to aromatic compounds, such as benzene and its derivatives, to effectively utilize lignin as the feedstock for bulk and fine chemicals [3] , [4] . Currently, heterogeneous catalysts play a major role in the hydrodeoxygenation of lignin-model compounds such as arenols and their ethers; however, the complete hydrogenation of the aromatic rings into saturated hydrocarbons over the catalyst surface was mostly inevitable under these conditions [7] . Thus, the preconversion of arenols to more activated esters was essential for the selective hydrogenolysis of the aryl–oxygen bonds over hydrogenation of the aromatic rings [8] . Recently, a few examples have been reported for the selective reductive cleavage of the less activated aryl–oxygen bonds in the alkyl ethers of arenols using either heterogeneous catalysts [4] , homogeneous nickel catalysts with a phosphine or a carbene ligand [9] , [10] , [11] , [12] , iron catalysts [13] or Lewis bases [14] . It should be noted, however, that none of the reported catalysts were applicable to the selective hydrodeoxygenation of free arenols, which would enable the complete deoxygenation of arenols to simple aromatic chemicals. To solve the problem, we envisioned a strategy utilizing the cooperative activation of arenols using hydroxycyclopentadienyl hydrido metal complexes, as shown in Fig. 1 : a cyclopentadienone–metal species, which was reported to cleave the H–H bond of dihydrogen heterolytically [15] , [16] , reacts with dihydrogen, affording a hydroxycyclopentadienyl hydrido metal complex. If the proton on the ligand and the hydride on the metal are delivered to an arenol in a concerted manner, the sp 2 C–OH bond in an arenol would be cleaved into an arene and water. 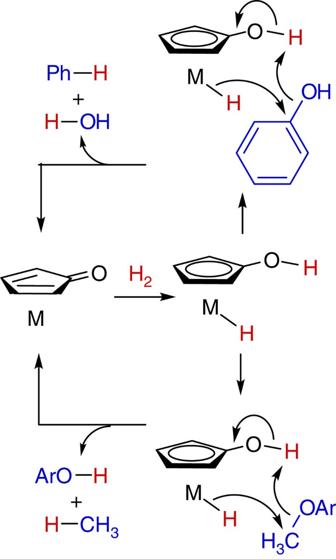Figure 1: Hydrogenolysis of arenols and aryl methyl ethers via metal–ligand cooperative hydrogen transfer. Dihydrogen is split into a proton on the hydroxycyclopentadienyl ligand and a hydride on the metal, which are transferred to a C–O single bond in a concerted manner. Figure 1: Hydrogenolysis of arenols and aryl methyl ethers via metal–ligand cooperative hydrogen transfer. Dihydrogen is split into a proton on the hydroxycyclopentadienyl ligand and a hydride on the metal, which are transferred to a C–O single bond in a concerted manner. Full size image Here in this communication, we report direct and selective hydrogenolysis of sp 2 C–OH bonds in arenols by hydroxycyclopentadienyl dihydridoiridium catalysts. Hydrogenolysis of sp 3 C–O bonds in aryl methyl ethers were also achieved using the same catalysts. These catalyses were further applied to deoxygenation of a lignin model compound, implying the potential application for mass production of arenes from lignin or its degraded components. Hydrogenolysis of sp 2 C–OH bonds in arenols The hydrogenolysis reactions of the sp 2 C–OH bond in phenols and naphthols were accomplished using hydroxycyclopentadienyl iridium complexes A and C as the catalysts under 1 atm of dihydrogen pressure at 200 °C ( Table 1 ; Fig. 2 ). From para -phenylphenol, biphenyl was obtained in 57% yield using the iridium complex A (entry 1). The reaction was strongly suppressed with complex B , a silyl-protected analogue of complex A , indicating that the free hydroxy group plays an important role in this catalysis (entry 2). Most probably, in entry 2, the catalysis was mediated by the species desilylated under the reaction conditions (see Supplementary Fig. 4 and Supplementary Discussion ). Triphenylphosphine complex C showed a higher activity than the di- tert -butylmethylphosphine complex A , affording biphenyl in 91% yield (entry 3). In sharp contrast to the results obtained using iridium complexes A and C , no reaction was observed with Cp* iridium complex D without the hydroxy group, or with ruthenium catalyst E , a ruthenium analogue of A , a combination of Ni(cod) 2 and N , N ′-(2,6-diisopropylphenyl)imidazolinylidene (SIPr) ( F ), which was effective for the hydrogenolysis of sp 2 C–OMe bonds, did not show any activity either ( Supplementary Table 1 ) [9] . This reaction was sensitive to steric demand, and the yield of biphenyl was strongly affected by the position of the phenyl substituent. A comparison among the para -, meta - and ortho -substrates indicated that the reactivity decreases in this order (entries 4 and 5). Notably, 1- and 2-naphthols could be successfully converted to naphthalene along with the formation of minimal amounts of 1,2,3,4-tetrahydronaphthalene, a side product resulting from over-reduction. The reaction was never achieved by either heterogeneous or homogeneous catalysts, before; this is because in all the cases, the hydrogenation of the aromatic rings dominated over the C–O bond cleavage [17] , [18] . Thus, both with catalysts A and C , the complete consumption of 1- or 2-naphthol was observed (entries 6–9). From 2-naphthol, naphthalene was obtained as the sole product in excellent yields (98% and 99%, entries 6 and 7, respectively), whereas the reactions of 1-naphthol afforded 17–23% of 1,2,3,4-tetrahydronaphthalene as a side product (entries 8 and 9). In entry 7, almost quantitative formation of water (91%) was confirmed by Karl Fisher titration. The reactions of naphthalenediols were either stopped on formation of naphthols (entries 10 and 12) or on conversion to naphthalene (entries 11 and 13) by changing the catalyst. The selectivity for the mono-deoxygenated product by complex A may have resulted from the catalyst deactivation during the reaction. (Please see Supplementary Figs 2–7 and Supplementary Table 1 for further experimental results.) Table 1 Hydrogenolysis of hydroxyarenes by iridium complexes*. 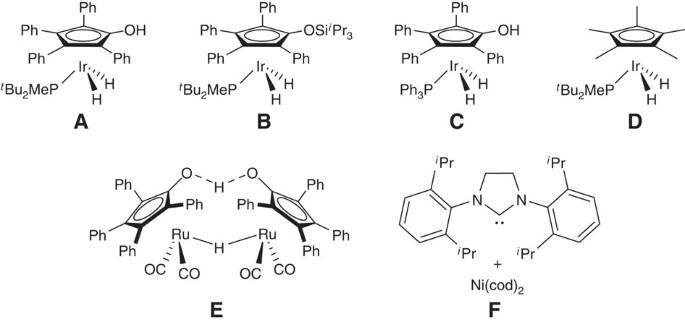Figure 2: Structures of catalysts. The figure shows molecular structures of the catalysts examined in this study. Full size table Figure 2: Structures of catalysts. The figure shows molecular structures of the catalysts examined in this study. Full size image Hydrogenolysis of sp 3 C–O bonds in aryl methyl ethers To our surprise, the selective hydrogenolysis of the sp 3 C–O bond, namely, demethylation, proceeded when 4-phenylphenyl methyl ethers and naphthyl methyl ethers were treated with hydroxycyclopentadienyl iridium dihydrido complexes A and C . For the demethylation of methyl ethers, that is, the deprotection of arenols, strong acids such as BBr 3 , AlCl 3 and trimethylsilyl iodide or basic nucleophiles such as NaSEt are usually used [19] . Although the metal-catalysed hydrogenolysis of the sp 3 methyl–oxygen bond in aryl methyl ethers would be an ideal candidate for a more atom-economical transformation under neutral conditions, all the preceding reduction reactions by transition metal catalysts resulted in the cleavage of sp 2 C–O bonds, but not sp 3 C–O bonds while only two exceptions were reported in a stoichiometric reaction with nickel(II) and iridium(0) [9] , [10] , [11] , [12] , [13] , [20] , [21] . The reaction also provides a new strategy for the production of arenols from lignin or its shorter fragments. With catalysts A and C , the hydrogenolysis of 4-methoxybiphenyl proceeded, affording 4-phenylphenol ( Table 2 , entries 1–4). In entry 3, the formation of methane was observed by gas chromatography (GC) analysis, proving that the demethylation reaction proceeds via the hydrogenolysis reaction. The reaction was significantly decelerated either in the absence of dihydrogen or in the presence of a small amount of water, both of which strongly supported that the reaction is not a simple hydrolysis reaction, but a hydrogenolysis reaction. Table 2 Hydrogenolysis of aryl methyl ethers by iridium complexes A and C*. Full size table We applied the hydrodeoxygenation/demethylation process to a model compound of lignin, vanillylacetone [2] ( Table 2 , entry 7). Vanillylacetone has three different types of oxygen functionalities, a phenolic hydroxy group, a methyl ether functionality and an aliphatic keto carbonyl group as the representative oxygen component of lignin and its degraded materials. When vanillylacetone was treated with 20 mol% of catalyst C under 1 atm of dihydrogen atmosphere for 50 h, completely deoxygenated butylbenzene and cyclized methyl indane were obtained as the two major products in 78% and 9% yields, respectively, while the yield of butylcyclohexane, a side product resulting from over-reduction, was suppressed to as low as 13%. Thus, the hydrodeoxygenation reaction successfully proceeded for phenolic C–OH bonds, aryl methyl ethers and aliphatic ketones in this lignin model compound (please see Supplementary Table 2 and Supplementary Figs 8 and 9 for further experimental results). The unique reactivity and selectivity in C–O bond hydrogenolysis, here we discovered with complexes A and C , may be explained by the catalytic cycles shown in Figs 3 and 4 . The mechanisms are still speculative at this moment. Shown in Fig. 3 is a proposed mechanism for the hydrogenolysis of sp 2 C–O bond in phenols. The starting dihydrido complex 1 is stabilized with two hydrogen bonds with one phenol molecule ( 1′ ). From phenol-stabilized complex 1′ , cleavage of a weak H–H bond provides intermediate 2, which undergoes outer-sphere transfer of a proton on the ligand and a hydride on the metal centre to a C–OH bond in a concerted manner via TS(2–3) . The mechanism is similar to the one proposed for the hydrogenation of carbonyl compounds by Shvo’s ruthenium catalyst E [15] . The successive heterolytic cleavage of dihydrogen assisted by one phenol molecule would afford complex 1′ . 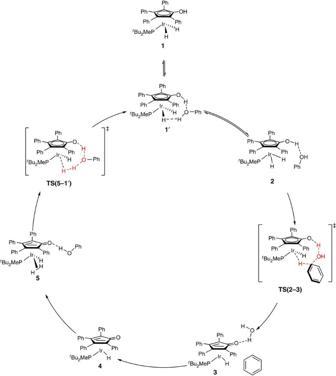Figure 3: Proposed mechanism for the hydrogenolysis of phenol. The proposed catalytic cycle for hydrogenolysis of phenol is shown. From dihydrido complex, C–O bond in phenol is cleaved via concerted proton and hydride transfer from ligand and iridium (TS2-3) to afford monohydrido complex4. Heterolytic dihydrogen split mediated by phenol affords the dihydrido complex (TS(5–1′)). Figure 3: Proposed mechanism for the hydrogenolysis of phenol. The proposed catalytic cycle for hydrogenolysis of phenol is shown. From dihydrido complex, C–O bond in phenol is cleaved via concerted proton and hydride transfer from ligand and iridium ( TS2-3 ) to afford monohydrido complex 4 . Heterolytic dihydrogen split mediated by phenol affords the dihydrido complex ( TS(5–1′) ). 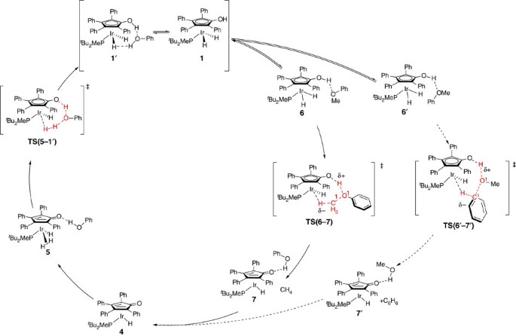Figure 4: Proposed mechanism for the hydrogenolysis of phenyl methyl ether. Proposed catalytic cycle for hydrogenolysis of sp3C–O bonds (viaTS(6–7)) and sp2C–O bonds (viaTS(6′–7′)) in anisole are shown. In both pathways, proton and hydride were delivered to C–O bonds in a concerted manner followed by heterolytic cleavage of dihydrogen mediated by phenol molecule (TS(5–1′)). Full size image Figure 4: Proposed mechanism for the hydrogenolysis of phenyl methyl ether. Proposed catalytic cycle for hydrogenolysis of sp 3 C–O bonds (via TS(6–7) ) and sp 2 C–O bonds (via TS(6′–7′) ) in anisole are shown. In both pathways, proton and hydride were delivered to C–O bonds in a concerted manner followed by heterolytic cleavage of dihydrogen mediated by phenol molecule ( TS(5–1′) ). Full size image For the hydrogenolysis of phenyl methyl ether, both the sp 2 and sp 3 C–O bond cleavages should be considered to reveal the reason why hydroxycyclopentadienyl iridium complexes A and C show the sp 3 C–O bond-selective cleavage, which is in contrast to the sp 2 C–O bond-selective cleavage reported for low-valent nickel or iron complexes ( Fig. 4 ) [9] , [10] , [11] , [12] , [13] . The outer-sphere dihydrogen transfer would prefer sp 3 C–O bond cleavage via 6 → 7 to sp 2 C–O bond cleavage via 6′ → 7′ . In the transition state for sp 3 C–O bond cleavage ( TS(6–7) ), we are now assuming the hydride on the iridium centre approaches the σ*-orbital of the sp 3 C–O bond in aryl methyl ether to undergo the S N 2 reaction. On the other hand, in the transition state for sp 2 C–O bond cleavage ( TS(6′–7′) ), the hydride approaches the π* orbital to make C 1 atom have sp 3 hybridization, causing the loss of aromaticity of the benzene ring in the transition state. In conclusion, the direct and selective hydrogenolysis of the sp 2 C–OH bonds in phenols and naphthols, and the selective hydrogenolysis of the sp 3 C–O bonds in aryl methyl ethers have been achieved using hydroxycyclopentadienyl iridium complexes A and C . A metal–ligand cooperative outer-sphere mechanism for the C–O bond cleavage was proposed to be responsible for the unique reactivity and selectivity of the reactions. The current chemical reduction technology has great potential for the future utilization of lignin as the chemical feedstock. General procedure for hydrogenolysis of arenols Into a 3-ml glass tube, catalyst (20 μmol) and substrate (200 μmol) were placed. The reaction vessel was connected to a rubber gas bag filled with dihydrogen and heated at 200 °C in a sand bath. After stirring at 200 °C for 20 h, a certain amount of dodecane (ca. 7.4 mg) was added as an internal standard and the products were analysed by GC. The products were also analysed by 1 H NMR analysis. Please see Supplementary Methods for further information. General procedure for hydrogenolysis of aryl methyl ethers Into a 3-ml glass tube, catalyst (1.0–20 μmol) and substrate (100 mg for solids, 200 μl for liquids) were placed. The reaction vessel was connected to a rubber gas bag filled with dihydrogen and heated at 200 °C in a sand bath. After stirring at 200 °C for the time indicated, a certain amount of dodecane (ca. 7.4 mg) was added as an internal standard and the products were analysed by GC. The products were also analysed by 1 H NMR analysis. Please see Supplementary Methods for further information. How to cite this article: Kusumoto, S. and Nozaki, K. Direct and selective hydrogenolysis of arenols and aryl methyl ethers. Nat. Commun. 6:6296 doi: 10.1038/ncomms7296 (2015).